Back-illuminated photoelectrochemical flow cell for efficient CO2reduction 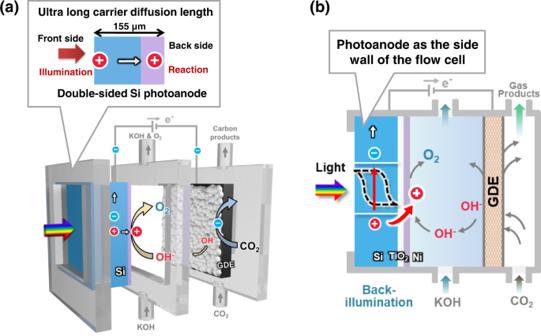Fig. 1: Si photoelectrode promoted flow cell. aThe schematic of the Si photoanode coupled flow cell with the gas diffusion electrode for PEC CO2RR.bThe cross-section of back-illuminated Si photoanode and the GDE cathode (figure not to scale for clarity). Photoelectrochemical CO 2 reduction reaction flow cells are promising devices to meet the requirements to produce solar fuels at the industrial scale. Photoelectrodes with wide bandgaps do not allow for efficient CO 2 reduction at high current densities, while the integration of opaque photoelectrodes with narrow bandgaps in flow cell configurations still remains a challenge. This paper describes the design and fabrication of a back-illuminated Si photoanode promoted PEC flow cell for CO 2 reduction reaction. The illumination area and catalytic sites of the Si photoelectrode are decoupled, owing to the effective passivation of defect states that allows for the long minority carrier diffusion length, that surpasses the thickness of the Si substrate. Hence, a solar-to-fuel conversion efficiency of CO of 2.42% and a Faradaic efficiency of 90% using Ag catalysts are achieved. For CO 2 to C 2+ products, the Faradaic efficiency of 53% and solar-to-fuel of 0.29% are achieved using Cu catalyst in flow cell. Photoelectrochemical (PEC) reduction of CO 2 use sunlight to directly drive the CO 2 RR for solar fuel production [1] , [2] , [3] . PEC CO 2 reduction systems, that utilize photocathode [4] , [5] and photoanode [6] , [7] driven systems, have been widely investigated. Photocathodes can employ CO 2 RRs catalysts to carry out the CO 2 RR in H-type cells, where the cell voltage could be supplemented by photovoltage, thus lowering the external energy input by photovoltage generated by photoelectrode [8] , [9] , [10] . However, many photocathodes suffer from low activity or poor stability for PEC CO 2 RR, because the catalyst/semiconductor interface tends to produce hydrogen and suffers from photo-corrosion in aqueous electrolytes [2] , [5] , [11] , [12] , [13] , [14] . Furthermore, the deployment of photocathodes in flow cell configurations for PEC CO 2 reduction remains a challenge because most high-performance semiconductor materials exist as dense layers, for which a compact substrate is always needed. Thus, it is a great challenge to simultaneously use semiconductors as a gas diffusion layer and sunlight absorber. On the other hand, photoanodes such as TiO 2 [15] , [16] , WO 3 [7] , BiVO 4 [7] , [17] , GaAs [18] , and Si [19] have been integrated to form PEC CO 2 reduction cells, and exhibit a reduced cell voltage for CO 2 reduction. However, there is still room to increase the current density, because many photoanode-assisted PEC CO 2 RR were all carried out in H-type cell [20] , [21] . The photoanode promoted flow cell for PEC CO 2 reduction is a promising way to improve the energy utilization efficiency. One of the prerequisites for flow cell photoelectrode operation is for the photoelectrode to generate a significant photocurrent, allowing the reduction reaction to proceed at a high rate. Irtem et al. elegantly pioneered a TiO 2 photoanode-assisted flow cell for the reduction of CO 2 to HCOO − , which demonstrated the feasibility of employing photoelectrodes within flow cells [22] . In this configuration, however, only photoanodes with wide bandgaps such as TiO 2 [23] , [24] , Fe 2 O 3 [25] , WO 3 [26] , BiVO 4 [27] , etc. could only be used since light could be introduced from the back side of the photoanode through the FTO substrate, leaving the front side facing the cathode for reaction. The relatively small photocurrent density of wide bandgap photoanodes limits the reaction rate and changes the CO 2 reduction product distribution. Therefore, photoelectrodes capable of generating high photocurrents are highly desired for PEC CO 2 RR flow cells. Silicon (Si), a narrow bandgap photoabsorber, is a promising photoanode candidate to drive the PEC CO 2 RR in flow cells due to its high saturation current density (larger than 40 mA/cm 2 ) [4] , [28] , [29] , [30] , [31] . Moreover, single-junction Si solar cells are cheaper and have simpler fabrication processes than multi-junction solar cells designed for outer space applications [18] , [32] , [33] . However, most conventional Si photoanodes operate in the front-illumination mode (where illumination occurs on the same side as the catalysts and junction) because of its opaque nature, which makes it difficult to introduce light from its back side, and thus cannot be adapted to flow cell configurations [34] , [35] , [36] . Si with back-illuminated configurations is an elegant solution to this conundrum, as they decouple the location of light absorption and surface reaction sites [37] , [38] , [39] . Therefore, the implementation of back-illuminated Si photoelectrodes into PEC CO 2 RR flow cells has the potential to improve their energy utilization efficiency. This paper describes the design and realization of a PEC CO 2 RR system that integrates a Si-based narrow bandgap photoelectrode to convert solar energy into chemicals at high photocurrent densities. The light absorption and catalytic sites could be separated onto different sides of the opaque Si photoelectrode, eliminating the tradeoff between optimized light absorption and efficient CO 2 reduction in flow cells. The Si photoelectrode-assisted flow cell affords a high Faradaic efficiency of 90% and 53% for CO or C 2+ products respectively, achieving the solar-to-fuel (STF) conversion efficiency of 2.42% for CO products. This work provides a promising design strategy for Si-based solar fuel production. Configuration of PEC flow cell for CO 2 RR with a double-sided Si photoanode To realize a PEC flow cell for CO 2 RR, a Si photoelectrode integrated flow cell was proposed for CO 2 RR (Fig. 1a ). The left sidewall of the flow cell is the Si compartment, where water oxidation reaction (OER) takes place. Incident light was irradiated from the chamber with the open-hole plate, allowing the Si to absorb the light directly. The surface of Si was textured to micro-pyramid (Fig. S1 ) to decrease the surface reflectance (Fig. S2 ). The GDE was situated on the opposite of the Si compartment, to facilitate CO 2 RR. Various catalysts can be deposited onto the GDE for different kinds of CO 2 reduction products. Fig. 1: Si photoelectrode promoted flow cell. a The schematic of the Si photoanode coupled flow cell with the gas diffusion electrode for PEC CO 2 RR. b The cross-section of back-illuminated Si photoanode and the GDE cathode (figure not to scale for clarity). Full size image To construct a decoupled Si photoanode in which its illumination and catalytic sites are located on different sides and enable light absorption from the back side (Fig. 1b ), amorphous Si was deposited as passivation layer to saturate the dangling bonds on Si surface due to its superior chemical passivation effect (prepared by plasma enhanced chemical vapor deposition (PECVD), details in Methods) [28] . The amorphous Si passivated the Si substrate, exhibiting an ultra-high minority carriers lifetime (3275 μs) (Fig. S3 ), and long minority carrier diffusion length of 2015 μm (calculation details in the Methods). This ultra-long minority carrier diffusion length is much longer than the thickness of Si wafer (155 μm), enabling photogenerated minority carriers (holes) to move from one side of Si electrode to other side before recombining (Fig. 1a ). Thus, light absorption and surface reaction can be decoupled by having the light illumination side and OER catalyst layer on be located on different sides of Si substrate. Furthermore, two doped thin films (p type and n type amorphous Si) were deposited on amorphous Si (prepared by PECVD, details in Methods) to construct a built-in electric field to enhance the driving force for photogenerated carriers (Fig. S4 ). To evaluate the performance and stability of back-illuminated Si photoanode for water oxidation. 10 nm TiO 2 protective layer was deposited by atomic layer deposition (ALD). The thickness of TiO 2 was optimized to 10 nm in our previous work [40] , as the thickness presents no significant effect on the stability of the silicon photoanode for water oxidation when the thickness exceeds 8 nm [41] . Then 5 nm Ni with a larger surface-active area compared to thick Ni thin films deposited by direct current (DC) sputtering on TiO 2 as OER catalyst for Si photoanodes (photograph of Si photoanode in Fig. S5 ). The back-illuminated Si photoanodes exhibit a dense surface morphology after TiO 2 and Ni deposition (Fig. S7 ). For PEC measurements, the Si photoanode was evaluated under AM 1.5 G illumination (100 mW/cm 2 ). To be consistent, 1 M KOH (pH 13.7) was used as the CO 2 RR in flow cell electrolyte [42] . The Si photoanode showed an early onset potential of 0.8 V vs. reversible hydrogen electrode (RHE) and high saturation photocurrent density (38 mA/cm 2 ) (Fig. 2a ), a significantly reduced onset potential compared with electrochemical OER. This photocurrent density is also much higher than that of wide band-gap photoelectrodes (smaller than 5 mA/cm 2 ), demonstrating the merits of narrow band-gap photoelectrode for CO 2 RR in flow cells. The photogenerated voltage of this back-illuminated Si photoanode, determined by the difference in onset potential between the Si photoanode and degenerated p + -Si/TiO 2 /Ni electrode with no photo response (Fig. 2a ), was about 700 mV at current density comprised between 1 and 38 mA/cm 2 , as indicated. Holes were the majority and minority carriers of the p + -Si/TiO 2 /Ni dark electrodes, respectively. To fairly compare surface reactions between the Si dark electrode and photoelectrode, the TiO 2 protective layer and Ni catalyst layer of dark electrodes were prepared under same batch as Si photoanode (Fig. S8 ). A high applied bias photon-to-current efficiency (ABPE) of 5.4% was obtained (Fig. 2b ). The high ABPE and stability can be attributed to the efficient light utilization efficiency achieved by the back-illumination structure. Furthermore, the stability of Si photoanodes was evaluated by a chronoamperometry test at a fixed applied potential of 1.5 V vs. RHE. The photocurrent remains stable for over 150 h (Fig. 2c ). The Faradaic efficiency of O 2 generation for Si photoanode is higher than 97% at 1.5 V vs. RHE under AM 1.5 G irradiation over a 150-h, indicating that most of the photogenerated holes are consumed for OER (Fig. 2c ). The surface morphology is nearly unchanged after the stability test (Fig. S7 ). Moreover, grazing incidence X-ray diffraction (GIXRD) patterns of Si photoanode showed similar ITO diffraction peak intensity before and after stability (Fig. S9 ). Ni catalyst layer was stabilized on the surface of TiO 2 by metal–support interaction [43] , and partially transformed to NiO x or NiOOH after stability test (Fig. S6 ). This robust stability is attributed to the ALD-deposited TiO 2 separating the electrolyte and Si photoanode, preventing corrosion. The superior activity and stability of this back-illuminated Si photoanode configuration have the potential to operate in flow cells with reduced cell voltage and improved energy utilization efficiency for CO 2 RR. Fig. 2: Performance of back-illuminated Si photoanode. a The current-voltage curves, b ABPE and c Time-dependent photocurrents (left-axis) and Faradaic efficiency toward O 2 (right-axis) under simulated AM 1.5 G illumination. Inset: Schematic of the light absorption and reaction decoupled Si photoanode. Full size image High-rate CO 2 reduction in PEC flow cell with controllable product distribution Benefiting from the back-illuminated configuration, this Si photoelectrode could be used as the photoanode for OER in the CO 2 RR flow cell. The CO products were generated using metallic Ag as the catalyst (photograph in Fig. S10a ) alongside our back-illuminated Si photoanode in flow cell with (photograph in Figs. S11 , S12 ). 50 nm Ag catalyst was deposited on carbon paper by DC sputtering (Fig. 3a ), which appeared to a continuous surface (Fig. S13 ). Ag catalyst is highly crystalline and shows a face-centered cubic crystal structure (Fig. S14 ). The CO 2 RR was carried out in 1 M KOH to suppress the hydrogen evolution, and the Si photoanode was performed under AM 1.5 G illumination (100 mW/cm 2 ). To verify the benefits of back-illuminated Si photoanode in lowering cell voltage, the current–voltage ( J – V ) curves of CO 2 RR were collected in a two-electrode configuration (Fig. 3b ). The back-illuminated Si photoanode promoted flow cell only required cell voltages as low as 1.44 V to obtain the current density of 10 mA/cm 2 , which is 720 mV lower than the conventional dark anode (p + -Si/TiO 2 /Ni) using Ni as the catalyst (2.16 V). This is consistent with the photovoltage of the back-illuminated Si photoanode (Fig. 2a ). Therefore, the external energy input for CO 2 RR was significantly decreased by the reduction OER energy consumption. The performance of the back-illuminated Si photoanode-assisted CO 2 RR to produce CO was evaluated over Ag catalysts at different current densities (Fig. 3c ), where the exclusive formation of gaseous CO and H 2 is observed in the gas phase. The Ag catalyst exhibited a selectivity of more than 90% for the reduction of CO 2 to CO under wide current density range of 3–38 mA/cm 2 (Fig. 3c ), which is consistent with previously reported results in electrochemical CO 2 reduction [44] , [45] , [46] . Moreover, the durability of PEC flow cell for CO production was evaluated, where the FE of CO remained nearly unchanged throughout the test duration (Fig. 3d ). To further evaluate the stability of this Si electrode-promoted flow cell, p + -Si/TiO 2 /Ni was used as dark electrode (Fig. S8 ). The current density of dark electrode continuously decreased during the 10 h stability test, having the same trend of decline as the Si photoelectrodes (Fig. S17 ). J – V curves of p + -Si/TiO 2 /Ni dark electrodes show no degradation during its 10 h stability test (Fig. S16 ). However, the formation of carbonate on the GDE surface (photograph in Fig. 15 ) was shown to inhibit CO 2 transport and reduce the number of available catalytic sites after a 12 h stability test in dark (Fig. S17 ), leading to a decreased current density (Fig. 2c ) [47] , [48] . Furthermore, carbonation of the electrolyte tends to shift the pH towards the neutral regime (from 13.7 to 13.4), resulting in higher solution resistance and unfavorable kinetics for OER, consistent with former investigations [49] , [50] . Therefore, the increased cell voltage can be attributed to the formation of carbonate on the GDE and the decreased pH of electrolyte. Fig. 3: Performance of CO 2 to CO with Si photoanode assistance. a The schematic of Ag cathode. b The J – V curves of CO 2 RR with and without Si photoanode in a two-electrode configuration. c The FE of CO at different current densities. d Time-dependent photocurrents (left-axis) and FE toward CO (right-axis) under simulated AM 1.5 G illumination. Full size image In addition to CO, multi-carbon products with high energy densities such as C 2 H 4 and C 2 H 5 OH are also producible from this PEC flow cell configuration [20] , [51] . 100 nm Cu was sputtered on carbon paper GDE in this work (photograph in Fig. S10b ). X-ray diffraction and X-ray photoelectron spectroscopy confirmed the existence of metallic Cu (Figs. S18 , S19 ). The Cu catalyst was combined with the back-illuminated Si photoanode to carry out the CO 2 RR in flow cell using 1 M KOH (pH 13.7) as the electrolyte (Fig. 4a ) (photograph in Fig. S20 ). Fig. 4: Performance of CO 2 to C 2+ with Si photoanode assistance. a The schematic of Cu cathode. b The J – V curves of CO 2 RR with and without Si photoanode in a two-electrode configuration. c The FE of C 2+ at different potentials. d Time-dependent photocurrents (left-axis) and FE toward C 2+ (right-axis) under simulated AM 1.5 G illumination. Full size image Compared to the system without back-illuminated Si photoanodes, external the voltage input was lower by 700 mV in Si photoanode-assisted flow cell, indicating that the high photovoltage can be provided by the back-illuminated Si photoanode to produce multi-carbon products (Fig. 4b ). 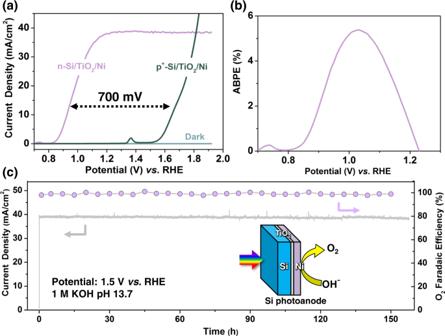Fig. 2: Performance of back-illuminated Si photoanode. aThe current-voltage curves,bABPE andcTime-dependent photocurrents (left-axis) and Faradaic efficiency toward O2(right-axis) under simulated AM 1.5 G illumination. Inset: Schematic of the light absorption and reaction decoupled Si photoanode. The FE for C 2+ products including C 2 H 4 , C 2 H 5 OH, and propanol reaches 53% on Cu catalysts, comparable to FE of unmodified metallic copper electrocatalysts (Fig. 4c ) [52] , [53] , [54] . Furthermore, the FE of C 2+ products reached 53% with the help of Si photoanode during its 5 h operation (Fig. 4d ). Therefore, the back-illuminated Si photoanode can feasibly be coupled with CO 2 RR flow cell operating at high reaction rates and maintain the same FE and stability as electrocatalytic CO 2 reduction flow cells. Energy conversion of PEC flow cell with Si photoelectrode The back-illuminated Si photoanode has been successfully coupled with the flow cell, and maintained a decent activity and stability for converting CO 2 to CO, C 2 H 4 and C 2 H 5 OH. The back-illuminated Si photoanode effectively reduced the energy consumed from the external electrical power supply. To assess the contribution of Si photoanode to the CO 2 reduction system, the STF conversion efficiency of the Si promoted cell was calculated by Eq. ( 1 ): 
    η_STF=∑(E^0-V_II)×I×FE/P_in× 100%
 (1) The thermodynamic potential of the respective product ( E 0 ) of CO, C 2 H 4 , C 2 H 5 OH, and C 3 H 7 OH are respectively equal to 1.334, 1.150, 1.147, and 1.131 V [20] , [51] . V II is the cell voltage measured in two electrodes (Figs. 3 b, 4b ). I is the operating current density at different voltages. FE is Faradaic efficiency for target product. P in is the input power (100 mW/cm 2 in this work). The active area of the Si photoanode was 1 cm 2 . For the conversion of CO 2 to CO, the FE of CO was larger than 90% in the voltage range of 0.3–1.334 V (Fig. 3b ), leading to a high STF efficiency of 2.42% (Fig. 5a ). To the best of our knowledge, this is the highest STF efficiency among photoanodes assisted cell for PEC CO 2 RR (Fig. 5b ), also surpassing the STF efficiency of state-of-the-art photocathodes for PEC CO 2 RR (Fig. 5b ). The STF for C 2+ products reaches 0.29% (Fig. S21 ), which is lower than that of CO because the generation of C 2 H 4 and C 2 H 5 OH (8 and 12 electrons reactions, respectively) is kinetically more difficult than the two-electron reduction products (CO) [20] , [54] . Although the STF efficiency in this work is lower than photoelectrodes fabricated from multi-junction III–V semiconductors under concentrated illuminations, the Si-based PEC flow cell holds the merit of low costs and facile fabrication processes [18] , [32] . Therefore, the Si photoanode could effectively reduce the high overpotential in OER, while maintaining a reasonable performance to produce CO 2 reduction to CO or C 2+ products compared with the conventional electrochemical CO 2 reduction in the flow cell. Fig. 5: Calculation and comparison of STF efficiency. a STF efficiency of PEC Si photoanode for the conversion of CO 2 to CO and b Performance comparison of photoanodes and photocathodes promoted cell for PEC CO 2 RR. Chart visualizing data on FE of products, photocurrent density, and STF for PEC CO 2 RR. Details are provided in Tables S1 , S2 . Full size image In summary, this paper demonstrates a PEC flow cell for CO 2 reduction with a back-illuminated Si photoanode that improves energy utilization efficiency. To overcome the contradiction between the opaque semiconductor light absorber and gas diffusion electrode in a flow cell, the Si photoelectrode was passivated by amorphous Si to obtain an ultra-long minority carrier diffusion length and separate the light absorption region from the catalytic sites. This decoupled structure enables the light to be introduced from the anode compartment side instead of the cathode side, when the photoanode is used as a sidewall of the cell. In this configuration, a high reaction rate (38 mA/cm 2 ) for CO 2 reduction was achieved in the PEC flow cell for CO 2 RR. For the conversion of CO 2 , the back-illuminated Si photoanode-assisted PEC flow cell shows an STF efficiency of 2.42% for CO with a FE of 90% using Ag catalyst. The direct PEC flow cell for CO 2 RR to C 2+ products is achieved at a FE of 53% on Cu catalyst and an STF of 0.29% is achieved. The design strategy in this work opens promising approaches based on Si photoelectrodes to generate solar fuels from CO 2 and H 2 O towards industrial application. Fabrication of Si photoelectrode with amorphous Si passivation layer Czochralski (CZ) c-Si wafers (n-type) with the resistivity of 1–5 Ω cm, 155 μm thickness and (100)-orientation were used as the substrate for Si electrode peparation. Silicon wafer was first textured using a mixture of potassium hydroxide (KOH) and isopropyl alcohol (IPA) (Top view SEM images in Fig. S1 ), then cleaned by standard RCA cleaning methods and finally dipped in 5% HF for 60 s to get rid of surface native oxide thin film. The Si wafer was then put into the PECVD chamber. 5 nm Intrinsic amorphous Si thin films were used to passivate the front and back side surfaces of Si substrate. n + amorphous Si and p + amorphous Si were deposited on the intrinsic amorphous Si (Fig. S4 ). WCT-120 lifetime tester from Sinton Instruments was applied for minority carrier lifetime test. Deposition of TiO 2 protective layer 10 nm of amorphous TiO 2 was deposited onto the above Si photoelectrodes at 150 °C in a custom-made ALD system, using Titanium (IV) isopropoxide (TTIP, Sigma-Aldrich, ≥99.9999%) and ultrapure water as precursors. The precursors were held at 70 °C and 25 °C, respectively. One ALD cycle consists of TTIP dose for 1 s, N 2 purge for 10 s, water dose for 0.1 s and N 2 purge for 10 s. The growth per cycle for TiO 2 is 0.3 Å/cycle. Deposition of Ni catalytic layer Ni was deposited by custom-made direct current magnetron sputtering. The sputtering target is Ni with high purity (99.99%). The chamber base pressure was kept at 10 −5 Pa, and then high-purity Ar flow was fed into the chamber. The gas flow was controlled at 20 sccm by mass flow controllers. The process pressure was fixed at 1 Pa and deposition time can be regulated to adjust the thickness of the film. Preparation of dark Si electrode Czochralski (CZ) p-type c-Si wafers with the resistivity of 0.001–0.005 Ω cm, 525 μm thickness and (100)-orientation were used as substrate. The ohmic back contacts were formed by rubbing the back side surfaces of the Si samples with a Ga–In alloy (99.9% metal basis, Alfa Aesar). PEC measurements PEC measurements were performed using a three-electrode configuration with Si electrode as the working electrode, Hg/HgO as the reference electrode in alkaline electrolyte. Schematic illumination and photograph of the apparatus used in the PEC measurement are shown in Fig. S22 . The potentials were converted into values against reversible hydrogen electrode using the Nernst Eq. ( 2 ) for dark cathode and photoanodes. V_RHE=V_Hg/HgO+0.098(V)+0.059pH
 (2) The potentiostat (CompactStat.e20250, IVIUM) was used to measure the J – V curves and chronoamperometry (without iR compensation). J – V curves of samples were measured with a scan rate of 50 mV s −1 under the irradiation of a 150 W xenon lamp (SAN-EI ELECTRIC CO., LTD) equipped with an AM 1.5 G filter. The active geometric areas of the working electrode were calibrated by the software Image J. 
    ABPEs=I× (1.23-V_b)/P× 100%
 (3) The applied bias photon-to-current efficiencies of photoanode were calculated using the J – V curves with an assumption of 100% Faradaic efficiency, according to Eq. ( 3 ). Where I (mA/cm 2 ) is the photocurrent density under an applied bias of V b (V vs. RHE), and P is the incident illumination intensity (mW/cm 2 ) (100 mW/cm 2 in this work). Analysis of CO 2 reduction products During electrolysis, the gas mass flow controller was set to 20 sccm, the peristaltic pump was set to 30 rpm (photograph in Fig. S23 ), gas products were quantified using an online gas chromatography system (GC7890B, Agilent Technologies, Inc.). H 2 , O 2 , and N 2 were detected by thermal conductivity detector (TCD) (MolSieve 5A packed column, Agilent Technologies, Inc.) and CO was detected by back-flame ionization detector (FID) (Porapak Q packed column, Agilent Technologies, Inc.). A methanizer was installed to enable the back FID to detect CO with 1000 times higher sensitivity. Ar was used as the carrier gas. After passing through the reactor, the gas was allowed to flow directly into the gas sampling loop of the gas chromatography for online gaseous product analysis. The Faradaic efficiencies of the gas products were calculated by using the concentrations (ppm) detected by the GC as following Eq. ( 4 ): 
    FE%=ppm×flow rate  (sccm)×nFp_0/RT/j_total  (mAcm^2)× 100%
 (4) Where n is the number of electrons transferred to CO 2 to produce a given product ( n (CO) = 2; n (C 2 H 4 ) = 12; n (C 2 H 5 OH) = 12), p 0 is the pressure (101.325 kPa) and T = 273.15 K, R is the gas constant (8.314 J mol –1 K –1 ). Characterization The thickness of amorphous Si, TiO 2 , Ni, Au and Ag layers on polished Si(100) monitor substrate was determined by spectroscopic ellipsometer (M-2000 DI, J.A. Woollam Co., Inc.) at 60° and 70° incident angle, by fitting the amplitude ratio ( Ψ ) and phase shift ( Δ ) of polarized light with the Cauchy dispersion model for a-Si and TiO 2 , and a tabulated metallic model for Ni, Au, and Ag. The morphology was carried out by field emission scanning electron microscope (FESEM, Hitachi S-4800, 5 kV). XPS analysis was conducted on a Physical Electronics PHI 1600 ESCA system with an Al Kα X-ray source (1486.6 eV). The binding energy was calibrated against the C 1 s photoelectron peak at 284.6 eV as the reference. The optical reflectance measurement of the Si was performed using spectrophotometer (Shimadzu UV-3600). The X-ray diffraction (XRD) (D/MAX-2500, Rigaku) spectra were collected over a 2 θ range from 20° to 80° at a scanning speed of 0.02° per step. 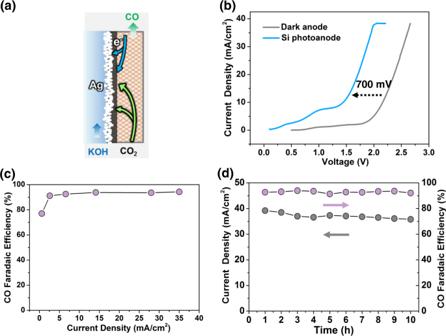Fig. 3: Performance of CO2to CO with Si photoanode assistance. aThe schematic of Ag cathode.bTheJ–Vcurves of CO2RR with and without Si photoanode in a two-electrode configuration.cThe FE of CO at different current densities.dTime-dependent photocurrents (left-axis) and FE toward CO (right-axis) under simulated AM 1.5 G illumination. Calculation of the minority carrier diffusion length 
    1/τ_eff=1/τ_bulk+2S/W
 (5) The surface recombination velocity can be calculated by Eq. ( 5 ) for the Si electrode with a-Si passivation, where W is the thickness of Si wafer, τ bulk is the bulk minority carrier lifetime, S is the surface recombination velocity. 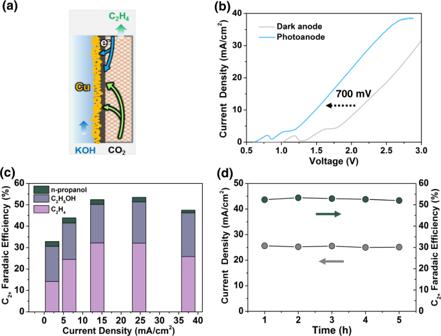Fig. 4: Performance of CO2to C2+with Si photoanode assistance. aThe schematic of Cu cathode.bTheJ–Vcurves of CO2RR with and without Si photoanode in a two-electrode configuration.cThe FE of C2+at different potentials.dTime-dependent photocurrents (left-axis) and FE toward C2+(right-axis) under simulated AM 1.5 G illumination. 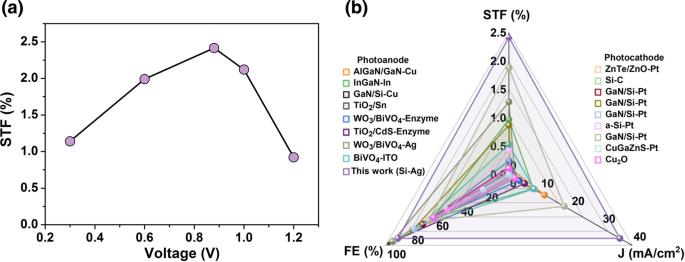Fig. 5: Calculation and comparison of STF efficiency. aSTF efficiency of PEC Si photoanode for the conversion of CO2to CO andbPerformance comparison of photoanodes and photocathodes promoted cell for PEC CO2RR. Chart visualizing data on FE of products, photocurrent density, and STF for PEC CO2RR. Details are provided in TablesS1,S2. L_p=√(τ_pD_p)
 (6) The minority carrier diffusion length of Si photoelectrode can be calculated by Eq. ( 6 ), where τ p is the minority carrier lifetime of n-type Si, D p is the diffusion coefficient of hole ( D p = 12.4 cm 2 /s, at 298 K) [55] , [56] .